Dll1 maintains quiescence of adult neural stem cells and segregates asymmetrically during mitosis Stem cells often divide asymmetrically to produce one stem cell and one differentiating cell, thus maintaining the stem cell pool. Although neural stem cells (NSCs) in the adult mouse subventricular zone have been suggested to divide asymmetrically, intrinsic cell fate determinants for asymmetric NSC division are largely unknown. Stem cell niches are important for stem cell maintenance, but the niche for the maintenance of adult quiescent NSCs has remained obscure. Here we show that the Notch ligand Delta-like 1 (Dll1) is required to maintain quiescent NSCs in the adult mouse subventricular zone. Dll1 protein is induced in activated NSCs and segregates to one daughter cell during mitosis. Dll1-expressing cells reside in close proximity to quiescent NSCs, suggesting a feedback signal for NSC maintenance by their sister cells and progeny. Our data suggest a model in which NSCs produce their own niche cells for their maintenance through asymmetric Dll1 inheritance at mitosis. The adult mammalian brain contains neural stem cells (NSCs) that generate neurons and glial cells throughout the lifetime of an organism. NSCs reside in at least two regions of the adult brain, the subventricular zone (SVZ) of the lateral ventricles and the subgranular zone of the hippocampus. Newborn neurons are incorporated into the existing functional networks and are thought to have important innate and adaptive roles in cognition, behaviour and tissue repair [1] , [2] , [3] . A fundamental question relevant to the ‘stemness’ of adult NSCs concerns how the pool size of this population is maintained over long periods while continuously producing neurons. In the adult SVZ, a subset of glial fibrillary acidic protein (GFAP)-expressing cells (type B cells) are relatively quiescent NSCs that are activated and produce their progeny [4] . Quiescence (or a low proliferation rate) is a common characteristic of a variety of adult tissue stem cells and is thought to contribute to long-term maintenance of the stem cell pool by preventing exhaustion of the limits of proliferation capacity or by reducing the probability of accumulating mutations [5] , [6] , [7] . Therefore, identifying the mechanism that regulates the quiescent state of adult NSCs is key to understanding how the adult stem cells are maintained. The maintenance and differentiation of stem cells are in general regulated by specialized local microenvironments known as niches [8] . Although previous studies have revealed some essential niches such as endothelial cells, ependymal cells and astrocytes to support the activation and differentiation of NSCs in the adult SVZ [9] , [10] , [11] , niche signals and niche cells responsible for the maintenance of quiescent NSCs (which inhibit NSC activation and differentiation) have been incompletely identified [1] , [12] , [13] , [14] , [15] , [16] . Another mechanism to maintain the stem cell pool is asymmetric cell division that produces one stem cell and one differentiating cell. This type of asymmetric cell division guarantees the maintenance of the stem cell at each mitosis in contrast to stochastic differentiation, which may risk the loss of the stem cell. Although NSCs have been proposed to undergo asymmetric cell division on the basis of studies of invertebrates [17] and of molecules that localize asymmetrically during or after mammalian NSC division—such as Par3, TRIM32 and the epidermal growth factor receptor (EGFR) in embryonic neocortical NSCs, as well as Dryk1 and EGFR in adult NSCs [18] , [19] , [20] , [21] —the identity and regulation of cell fate determinants that are asymmetrically distributed during mitosis in mammalian NSCs have only just begun to be elucidated. The Notch signalling pathway is highly conserved and is involved in stem cell maintenance in many systems [22] . Notch signalling is highly active in quiescent NSCs in the adult SVZ and subgranular zone, and it has a pivotal role in maintaining the undifferentiated and quiescent state of NSCs [12] , [23] , [24] , [25] , [26] , [27] , [28] , [29] . In the adult zebrafish telencephalon, it is also suggested that activated NSCs can be reversed to the quiescent state by Notch activation [30] . Notch is a transmembrane receptor that is activated by cognate ligands presented by neighbouring cells, and thus mediates signalling generated by cell–cell interaction ( trans activation) [31] . Ligand binding triggers cleavage of the intracellular domain of Notch (NICD), which then translocates to the nucleus and activates the transcription factor RBPJ, which in turn induces the expression of Hes genes and thereby suppresses the expression of proneural genes such as that for Ascl1 (also known as Mash1 ) [27] . Cells that express Notch ligands may therefore provide a niche for NSC maintenance through Notch activation. The Notch ligands Delta-like 1 (Dll1) and Jagged1 are expressed in the adult SVZ [23] , [32] , [33] , [34] . Which Notch ligands are responsible for the activation of Notch in NSCs and the maintenance of quiescent NSCs within the adult SVZ has remained unclear. Here we show that cells expressing the Notch ligand Dll1 reside in close proximity to quiescent NSCs in the SVZ of adult mice. Conditional deletion of the Dll1 gene in the adult SVZ results in a decrease in the number of cells manifesting Notch activation, as well as a decrease in the number of quiescent NSCs and an increase in that of activated NSCs, transit-amplifying cells and differentiating neuroblasts. Dll1 is expressed exclusively in activated NSCs and transit-amplifying cells, suggesting that NSCs begin to express Dll1 upon activation and that their progeny cells send a local feedback signal to support quiescent NSC maintenance. Unexpectedly, we find that Dll1 segregates asymmetrically during mitosis of NSCs in the adult SVZ as well as in the embryonic telencephalon. Time-lapse imaging of embryonic neocortical slice cultures and adult SVZ cultures reveals that enhanced green fluorescent protein (EGFP)-tagged Dll1 moves to one daughter cell during NSC mitosis, and that this Dll1-inheriting cell undergoes differentiation, whereas the cell that does not inherit Dll1 remains undifferentiated. These results suggest that NSCs give rise to their own niche cells through asymmetric segregation of Dll1 at mitosis, a process that may contribute to the ‘initialization’ of an activated NSC back to the basal (undifferentiated and quiescent) state of NSC. Dll1-positive cells reside in proximity to quiescent SVZ NSCs The activation of Notch signalling in adult NSCs would be expected to require their interaction with cells expressing a Notch ligand. Given that Dll1 is a major ligand for Notch activation in NSCs of the embryonic telencephalon [35] , we examined whether Dll1-expressing cells also make contact with NSCs in the adult SVZ. Slowly dividing (or quiescent) adult NSCs can be detected as label-retaining cells (LRCs) after pulse-chase treatment with a nucleotide analogue such as iododeoxyuridine (IdU) [4] , [36] . Immunohistofluorescence staining revealed that most (80.9±13.8%) LRCs in the SVZ of the adult mouse forebrain were positive for the active form of Notch (NICD) ( Fig. 1 ), confirming that Notch is activated in NSCs [12] , [26] . We found that Dll1 exhibited a characteristic punctate staining pattern, which is thought to reflect the active state of Notch ligand [37] , [38] , [39] , in a subset of SVZ cells in the adult mouse forebrain ( Fig. 1 ) (a movie of three-dimensional (3D) reconstruction from confocal images is shown in Supplementary Movie 1 ). The disappearance of Dll1-immunostaining puncta in Dll1-deleted brains ( Fig. 2a ) and the detection of Dll1-immunostaining puncta in most Dll1 -mRNA-expressing cells confirm the specificity of the antibody ( Supplementary Fig. S1 ). Using this antibody, we found that most (96.3±1.1%) of the Dll1 + cells were NICD negative ( Fig. 1 ). Importantly, Dll1 + cells were detected in close proximity (within a distance of 10 μm between nuclei) to most (84.4±7.2%) NICD + LRCs ( Fig. 1 ), suggesting that Dll1 might activate Notch in NSCs. 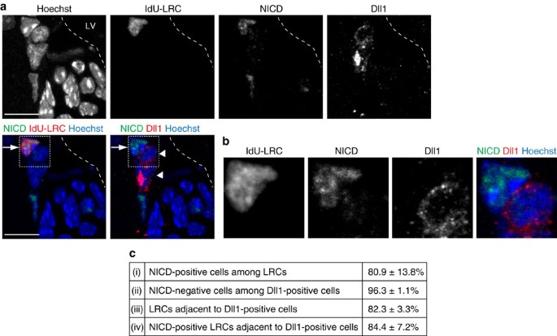Figure 1: Quiescent NSCs positive for activated Notch are located adjacent to Dll1-expressing cells in the adult mouse SVZ. Mice injected daily with IdU for 15 days were examined 21 days after the last injection. (a) Sections of the SVZ were subjected to immunofluorescence staining of IdU (for detection of LRCs), NICD and Dll1. Nuclei were stained with Hoechst 33342. LV, lateral ventricle. Arrows indicate NICD+IdU-LRCs, and arrowheads indicate Dll1+cells. Broken lines indicate the ventricular surface. (b) The boxed region inais shown at higher magnification. (c) The proportions of NICD+cells among LRCs (i), of NICD–cells among Dll1+cells (ii) and of LRCs (iii) or NICD+LRCs (iv) that were adjacent to Dll1+cells (within a distance of 10 μm between nuclei) are indicated (means±s.d.,n=3 brains). Total counted cells were LRCs=101 (i, iii), Dll1-positive cells=86 (ii) and NICD-positive LRCs=78 (iv). Scale bar, 10 μm. Figure 1: Quiescent NSCs positive for activated Notch are located adjacent to Dll1-expressing cells in the adult mouse SVZ. Mice injected daily with IdU for 15 days were examined 21 days after the last injection. ( a ) Sections of the SVZ were subjected to immunofluorescence staining of IdU (for detection of LRCs), NICD and Dll1. Nuclei were stained with Hoechst 33342. LV, lateral ventricle. Arrows indicate NICD + IdU-LRCs, and arrowheads indicate Dll1 + cells. Broken lines indicate the ventricular surface. ( b ) The boxed region in a is shown at higher magnification. ( c ) The proportions of NICD + cells among LRCs (i), of NICD – cells among Dll1 + cells (ii) and of LRCs (iii) or NICD + LRCs (iv) that were adjacent to Dll1 + cells (within a distance of 10 μm between nuclei) are indicated (means±s.d., n =3 brains). Total counted cells were LRCs=101 (i, iii), Dll1-positive cells=86 (ii) and NICD-positive LRCs=78 (iv). Scale bar, 10 μm. 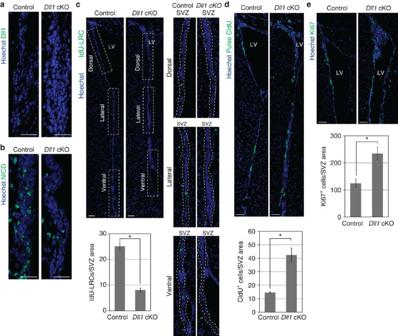Figure 2: Dll1 is required for maintenance of quiescent NSCs in the adult mouse SVZ. (a,b) Immunofluorescence staining of Dll1 (a) and NICD (b) in the SVZ of adult control (Dll1f/f) andDll1conditional knockout (cKO) (Dll1f/f;NesCreERT2) mice at 13 days after tamoxifen administration. Scale bar, 25 μm. (c) Control andDll1cKO mice were injected daily with IdU for 10 days. CreERT2 was then activated by tamoxifen administration, and the animals were examined 13 days thereafter. IdU-LRCs were detected by immunostaining, and the number of these cells in the SVZ was counted. The boxed regions (dorsal, lateral and ventral) in the upper left panels are shown at higher magnification in the right panels. Broken lines indicate the border of the SVZ. LV, lateral ventricle. Scale bar, 50 μm. Quantitative data are means±s.e.m. of values (the number of cells per 1 mm bin along the ventricular surface) from six sections of each brain. Total counted cells=202 (control), 71 (cKO). Student’st-test; *P<0.0001. (d) Control andDll1cKO mice were subjected to pulse (1 h) labelling with CldU at 13 days after tamoxifen administration, and rapidly dividing (CldU+) cells in the SVZ were detected by immunostaining and counted. Scale bar, 50 μm. Quantitative data are as inc. Total counted cells=117 (control), 375 (cKO). Student’st-test; *P<0.003. (e) Immunostaining of Ki67 in the SVZ of control andDll1cKO mice at 13 days after tamoxifen administration. Scale bar, 50 μm. Quantitative data are means±s.e.m. of values (the number of cells per 1 mm bin along the ventricular surface) from six sections of a control brain and eight sections of a cKO brain. Total counted cells=245 (control), 675 (cKO). Student’st-test; *P<0.002. Full size image Figure 2: Dll1 is required for maintenance of quiescent NSCs in the adult mouse SVZ. ( a , b ) Immunofluorescence staining of Dll1 ( a ) and NICD ( b ) in the SVZ of adult control ( Dll1 f/f ) and Dll1 conditional knockout (cKO) ( Dll1 f/f ;NesCreERT2) mice at 13 days after tamoxifen administration. Scale bar, 25 μm. ( c ) Control and Dll1 cKO mice were injected daily with IdU for 10 days. CreERT2 was then activated by tamoxifen administration, and the animals were examined 13 days thereafter. IdU-LRCs were detected by immunostaining, and the number of these cells in the SVZ was counted. The boxed regions (dorsal, lateral and ventral) in the upper left panels are shown at higher magnification in the right panels. Broken lines indicate the border of the SVZ. LV, lateral ventricle. Scale bar, 50 μm. Quantitative data are means±s.e.m. of values (the number of cells per 1 mm bin along the ventricular surface) from six sections of each brain. Total counted cells=202 (control), 71 (cKO). Student’s t -test; * P <0.0001. ( d ) Control and Dll1 cKO mice were subjected to pulse (1 h) labelling with CldU at 13 days after tamoxifen administration, and rapidly dividing (CldU + ) cells in the SVZ were detected by immunostaining and counted. Scale bar, 50 μm. Quantitative data are as in c . Total counted cells=117 (control), 375 (cKO). Student’s t -test; * P <0.003. ( e ) Immunostaining of Ki67 in the SVZ of control and Dll1 cKO mice at 13 days after tamoxifen administration. Scale bar, 50 μm. Quantitative data are means±s.e.m. of values (the number of cells per 1 mm bin along the ventricular surface) from six sections of a control brain and eight sections of a cKO brain. Total counted cells=245 (control), 675 (cKO). Student’s t -test; * P <0.002. Full size image Dll1 is necessary for maintenance of quiescent SVZ NSCs To investigate the necessity of Dll1 for the activation of Notch and the maintenance of NSCs in the adult SVZ, we conditionally deleted Dll1 in the adult brain by crossing mice with a floxed (f) Dll1 allele [40] with NesCreERT2 mice, in which a tamoxifen-responsive Cre (CreERT2) is expressed in adult NSCs in the SVZ under the control of a nestin promoter and enhancer [26] , [41] , [42] . Thirteen days after tamoxifen administration in adult Dll1 f/f ; NesCreERT2 ( Dll1 cKO) mice, the punctate pattern of Dll1 immunostaining in the SVZ had mostly disappeared ( Fig. 2a ), suggesting that Dll1 is expressed in NSC descendants. Importantly, the level of NICD immunostaining was also markedly reduced in the SVZ of Dll1 cKO mice ( Fig. 2b ), indicating that Dll1 is responsible for Notch activation in the adult SVZ. Because the number of Dll1-immunopositive cells appeared to be fewer than that of NICD + cells, it is possible that one Dll1-positive cell communicates with a number of adjacent NSCs to activate Notch signalling. We then examined the effects of Dll1 deletion on quiescent NSCs in the adult SVZ. Conditional ablation of Dll1 resulted in a significant decrease in the number of quiescent NSCs (LRCs) in the SVZ 13 days after tamoxifen treatment ( Fig. 2c ). Conversely, the number of rapidly dividing cells, detected either by pulse (1 h) labelling with chlorodeoxyuridine (CldU) ( Fig. 2d ) or by immunostaining for the cycling cell marker Ki67 ( Fig. 2e ), was increased. Next, we investigated the effects of Dll1 deletion on the lineage progression of adult NSCs. During lineage progression, quiescent NSCs (type B cells) (which are positive for GFAP and negative for EGFR) become activated (GFAP + EGFR + ) NSCs. They then produce GFAP – EGFR + Ascl1 + transit-amplifying cells (type C cells), which in turn give rise to neuroblasts (type A cells) positive for doublecortin (Dcx) and βIII-tubulin (TuJ1). We found that Dll1 deletion for 13 days did not significantly change the numbers of GFAP + cells and GFAP + Sox2 + double positive cells in the SVZ ( Fig. 3a ). These data indicated that the total number of NSCs is not affected by Dll1 deletion in this period. On the other hand, the number of activated NSCs, which were detected as GFAP + Ki67 + or GFAP + EGFP + cells, was significantly increased in the Dll1 -deleted SVZ ( Fig. 3b ). Dll1 deletion also increased the number of transit-amplifying cells (GFAP – EGFR + cells) ( Fig. 3c ) and, subsequently, that of neuroblasts (Dcx + or TuJ1 + cells) ( Fig. 3d ; data not shown). These results indicated that Dll1 has an essential role in the maintenance of quiescent NSCs within the adult SVZ, and abnormal activation of quiescent NSCs resulted in the increase of activated progeny. 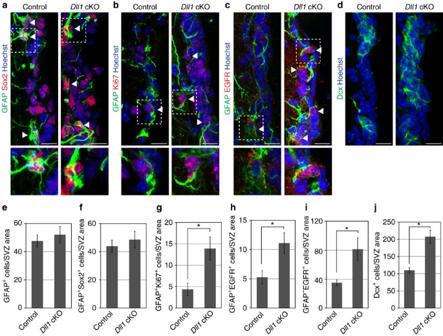Figure 3: Dll1 deletion increases activated progeny of quiescent NSCs in the adult mouse SVZ. (a–j) Immunostaining of GFAP with Sox2 (a), GFAP with Ki67 (b), GFAP with EGFR (c) and Dcx (d) in the SVZ of control andDll1cKO mice at 13 days after tamoxifen administration. Arrowheads indicate GFAP+Sox2+cells (a), GFAP+Ki67+cells (b) and GFAP+EGFR+cells (c). The boxed regions in the upper panels are shown at higher magnification in the lower panels. Scale bar, 10 μm. Quantitative data are means±s.e.m. of values (the number of cells per 1 mm bin along the ventricular surface) from eight sections of a control brain and six sections of a cKO brain (e–g), and from eight sections of a control brain and twelve sections of a cKO brain (h–j). Total counted cells were control=130 and cKO=105 (e), control=120 and cKO=98 (f), control=12 and cKO=28 (g), control=24 and cKO=56 (h), control=164 and cKO=389 (i), and control=507 and cKO=1068 (j). Student’st-test; *P<0.02 ing–i; *P<0.0005 inj. Figure 3: Dll1 deletion increases activated progeny of quiescent NSCs in the adult mouse SVZ. ( a – j ) Immunostaining of GFAP with Sox2 ( a ), GFAP with Ki67 ( b ), GFAP with EGFR ( c ) and Dcx ( d ) in the SVZ of control and Dll1 cKO mice at 13 days after tamoxifen administration. Arrowheads indicate GFAP + Sox2 + cells ( a ), GFAP + Ki67 + cells ( b ) and GFAP + EGFR + cells ( c ). The boxed regions in the upper panels are shown at higher magnification in the lower panels. Scale bar, 10 μm. Quantitative data are means±s.e.m. of values (the number of cells per 1 mm bin along the ventricular surface) from eight sections of a control brain and six sections of a cKO brain ( e – g ), and from eight sections of a control brain and twelve sections of a cKO brain ( h – j ). Total counted cells were control=130 and cKO=105 ( e ), control=120 and cKO=98 ( f ), control=12 and cKO=28 ( g ), control=24 and cKO=56 ( h ), control=164 and cKO=389 ( i ), and control=507 and cKO=1068 ( j ). Student’s t -test; * P <0.02 in g – i ; * P <0.0005 in j . Full size image Dll1 is expressed in the activated progeny of SVZ NSCs Given an essential role of Dll1 in the maintenance of quiescent NSCs, Dll1-expressing cells would be expected to serve as a niche that maintains this population. Different patterns of Dll1 expression in the adult SVZ have previously been described [23] , [32] , [34] . Using the anti-Dll1 antibody whose specificity was validated as mentioned above, we found that most Dll1 + cells in the SVZ of adult wild-type mice were positive for EGFR (88.8±3.8%) (total counted cells=219, n =3 brains), the transit-amplifying cell marker Ascl1 (78.7±7.3%) (total counted cells=143, n =3 brains) or the cycling cell marker Ki67 (81.0±5.3%) (total counted cells=184, n =3 brains) and were negative for the ependymal cell marker S100β (0%) (total counted cells=184, n =3 brains) or TuJ1 (7.8±3.6%) (total counted cells=145, n =3 brains) ( Fig. 4a ). Furthermore, 14.4±3.2% of Dll1-expressing cells were positive for both GFAP and EGFR (total counted cells=219, n =3 brains), and most (76.9±8.0%) activated NSCs (GFAP + EGFR + cells) were positive for Dll1 (total counted cells=46, n =3 brains) ( Fig. 4b ). These results suggested that activated NSCs and transit-amplifying cells express Dll1, and that these cells might serve as a niche that maintains quiescent NSCs in the adult SVZ. The size of the quiescent NSC pool in the SVZ might therefore be determined by a feedback signal elicited by the activated progeny of these cells. 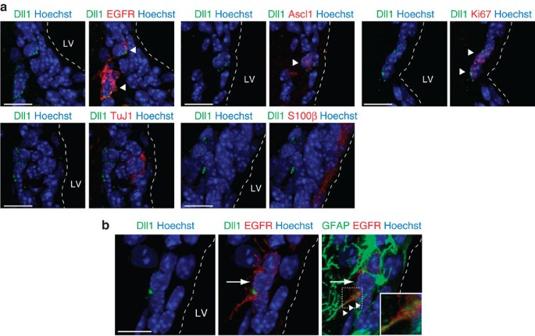Figure 4: Dll1 is expressed in activated NSCs and transit-amplifying cells in the adult mouse SVZ. (a) Immunofluorescence staining of Dll1 and the indicated markers in the adult SVZ. Arrowheads indicate cells positive for both Dll1 and the corresponding marker. Scale bar, 10 μm. (b) Detection of activated NSCs (GFAP+EGFR+cells) in the adult SVZ by immunofluorescence staining with antibodies to Dll1, GFAP and EGFR. Arrows indicate a Dll1+EGFR+GFAP+cell, and arrowheads indicate overlap between EGFR and GFAP staining in a process. The boxed region in the right panel is shown at higher magnification in the inset. Scale bar, 10 μm. LV, lateral ventricle. Broken lines indicate the ventricular surface. Figure 4: Dll1 is expressed in activated NSCs and transit-amplifying cells in the adult mouse SVZ. ( a ) Immunofluorescence staining of Dll1 and the indicated markers in the adult SVZ. Arrowheads indicate cells positive for both Dll1 and the corresponding marker. Scale bar, 10 μm. ( b ) Detection of activated NSCs (GFAP + EGFR + cells) in the adult SVZ by immunofluorescence staining with antibodies to Dll1, GFAP and EGFR. Arrows indicate a Dll1 + EGFR + GFAP + cell, and arrowheads indicate overlap between EGFR and GFAP staining in a process. The boxed region in the right panel is shown at higher magnification in the inset. Scale bar, 10 μm. LV, lateral ventricle. Broken lines indicate the ventricular surface. Full size image Dll1 is asymmetrically segregated at NSC mitosis The size of the NSC pool might also be maintained by asymmetric cell division that produces one stem cell and one committed or differentiated cell. However, cell fate determinants that segregate asymmetrically during mammalian NSC mitosis have remained largely unknown. Dll1 is implicated as a cell fate determinant of NSCs, given that it is an essential ligand for Notch activation in both embryonic [35] and adult (this study) NSCs within the forebrain and that it activates Notch in neighbouring cells (in trans ) and inactivates Notch within the same cell (in cis ) through direct binding and feedback loops [31] , [35] , [43] . We noticed that Dll1 was often asymmetrically distributed at mitosis in cultured NSCs prepared from the mouse neocortex (NCX) on embryonic day (E) 11.5 ( Fig. 5a ). We also found that a subpopulation (34.7±4.5% in NCX, 29.0±3.1% in ganglionic eminence (GE)) of phosphorylated vimentin-positive mitotic cells at anaphase–telophase manifested punctate Dll1 immunoreactivity at E14.5 embryonic telencephalon (total counted cells=245 (NCX), 165 (GE), n =3 brains). Remarkably, most (87.4±5.9% in NCX, 76.3±6.9% in GE) Dll1 + mitotic cells manifested asymmetric distribution of Dll1 at anaphase–telophase (total counted cells=85 (NCX), 48 (GE), n =3 brains) ( Fig. 5b ). 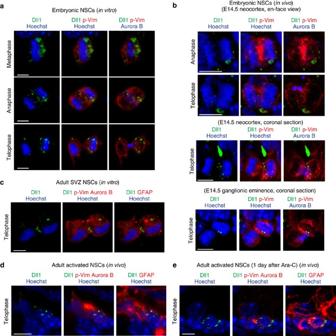Figure 5: Dll1 is asymmetrically segregated at NSC division. (a) Embryonic NSCs were prepared from neurosphere cultures of the mouse embryonic NCX at E11.5. The cells were subjected to immunofluorescence staining with antibodies to Dll1, phospho-vimentin (p-Vim) and Aurora B. Dll1+-dividing NSCs are shown. p-Vim and Aurora B are mitotic cell markers; Aurora B localizes to the central spindle at anaphase and to the midbody at telophase. Scale bar, 5 μm. (b) En-face views of the ventricular surface of the NCX, and coronal sections of the NCX and the GE of E14.5 mouse embryos stained as ina. Scale bar, 5 μm. (c) Adult SVZ NSCs were prepared from adult mouse SVZ. The cells were subjected to immunofluorescence staining with antibodies to Dll1, p-Vim, Aurora B and GFAP. Scale bar, 5 μm. (d,e) Divisions of activated NSCs (GFAP+divisions) in the SVZ of intact adult brain (d) or in the SVZ of adult brain at 1 day after treatment with Ara-C for 6 days (e). Sections were stained for Dll1, p-Vim, Aurora B and GFAP as indicated. The total numbers of divisions examined (anaphase–telophase) were 326 and 45, the numbers of GFAP+divisions among total divisions were 27/326 and 36/45, the numbers of Dll1+divisions among GFAP+divisions were 18/27 and 11/36, and the numbers of asymmetric Dll1 divisions among Dll1+GFAP+divisions were 15/18 and 11/11 fordande, respectively. These divisions were observed in a total of fifteen (d) and seven (e) brains. Scale bar, 5 μm. Figure 5: Dll1 is asymmetrically segregated at NSC division. ( a ) Embryonic NSCs were prepared from neurosphere cultures of the mouse embryonic NCX at E11.5. The cells were subjected to immunofluorescence staining with antibodies to Dll1, phospho-vimentin (p-Vim) and Aurora B. Dll1 + -dividing NSCs are shown. p-Vim and Aurora B are mitotic cell markers; Aurora B localizes to the central spindle at anaphase and to the midbody at telophase. Scale bar, 5 μm. ( b ) En-face views of the ventricular surface of the NCX, and coronal sections of the NCX and the GE of E14.5 mouse embryos stained as in a . Scale bar, 5 μm. ( c ) Adult SVZ NSCs were prepared from adult mouse SVZ. The cells were subjected to immunofluorescence staining with antibodies to Dll1, p-Vim, Aurora B and GFAP. Scale bar, 5 μm. ( d , e ) Divisions of activated NSCs (GFAP + divisions) in the SVZ of intact adult brain ( d ) or in the SVZ of adult brain at 1 day after treatment with Ara-C for 6 days ( e ). Sections were stained for Dll1, p-Vim, Aurora B and GFAP as indicated. The total numbers of divisions examined (anaphase–telophase) were 326 and 45, the numbers of GFAP + divisions among total divisions were 27/326 and 36/45, the numbers of Dll1 + divisions among GFAP + divisions were 18/27 and 11/36, and the numbers of asymmetric Dll1 divisions among Dll1 + GFAP + divisions were 15/18 and 11/11 for d and e , respectively. These divisions were observed in a total of fifteen ( d ) and seven ( e ) brains. Scale bar, 5 μm. Full size image We next examined the distribution of Dll1 puncta at mitosis in adult NSCs in vitro and in vivo . Similar to the embryonic NSCs, we found that Dll1 was asymmetrically segregated in dividing Dll1 + -activated NSCs (GFAP + phospho-vimentin + Aurora B + cells) in a culture of adult SVZ NSCs ( Fig. 5c ). Furthermore, we found that dividing Dll1 + -activated NSCs within the adult SVZ of fixed brains exhibited an asymmetric distribution of Dll1 (15/18 divisions (at anaphase–telophase), observed in 15 brains) ( Fig. 5d ) (a movie of the 3D reconstruction from confocal images is shown in Supplementary Movie 2 ). Given that quiescent NSCs rarely divide, we promoted the division of NSCs by treating mice with arabinosylcytosine (Ara-C). Treatment with Ara-C for 6 days eliminated most rapidly dividing cells such as transit-amplifying cells and neuroblasts (data not shown) [4] , [44] , [45] . At 1 day after such Ara-C exposure, when the division of NSCs was stimulated, the distribution of Dll1 at anaphase–telophase was again asymmetric in all the Dll1 + -activated NSCs (GFAP + divisions) examined (11/11 divisions (anaphase–telophase), observed in 7 brains) within the SVZ ( Fig. 5e ) (a movie of the 3D reconstruction from confocal images is shown in Supplementary Movie 3 ). These results indicated that Dll1 is asymmetrically segregated to one daughter cell at mitosis of activated NSCs in the adult SVZ, as well as during the division of embryonic neocortical NSCs. Dll1 might thus be a fate determinant that defines an asymmetric fate decision for the two daughter cells of an NSC. Dll1 protein moves to one daughter cell during NSC divisions Asymmetric cell division is often caused by an asymmetric environment that biases the fate of sister cells after cell division. Alternatively, a cell fate determinant might move to one sister cell intrinsically during cell division. To distinguish whether Dll1 asymmetry is established during or after cell division and to determine the fate of Dll1-inheriting daughter cells, we performed time-lapse imaging analysis in organotypic slice cultures. We observed the behaviour of EGFP-tagged Dll1 protein (Dll1-EGFP) during mitosis of NSCs present within embryonic neocortical slice cultures, because similar experiments are hard to perform with adult SVZ slices. Remarkably, time-lapse imaging revealed that most, if not all, Dll1-EGFP migrated to one daughter cell during mitosis (143 out of 157 Dll1 + divisions) ( Fig. 6a ; Supplementary Movie 4 ; also see Supplementary Fig. S2 ). Typically, Dll1-EGFP puncta were clustered around the central spindle and then moved to one daughter cell during anaphase, becoming dispersed within this daughter cell after telophase. We then examined the fate of the daughter cells that inherited or did not inherit Dll1-EGFP using immunohistofluorescence analysis after the time-lapse imaging. In most (9/10) asymmetric divisions that gave rise to one Tbr2 + neuronal progenitor and one Tbr2 − undifferentiated cell, the Tbr2 + cell inherited Dll1-EGFP ( Fig. 6b ; Supplementary Movie 5 ). The undifferentiated state of Tbr2-negative sister cells was confirmed on the basis of immunostaining for Sox2 or of cell position (in the ventricular zone) ( Supplementary Fig. S3 ). These results suggest that Dll1 inheritance is associated with neuronal differentiation. 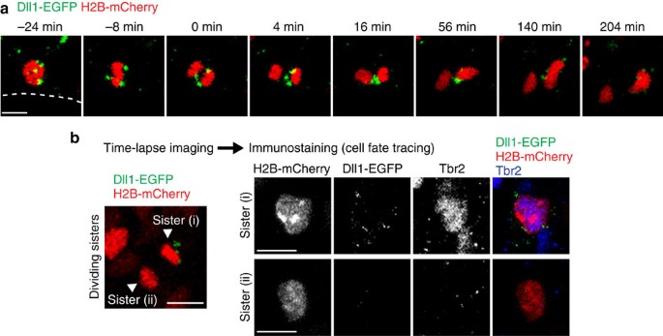Figure 6: Dll1-EGFP moves to one daughter cell that becomes a neuronal progenitor during asymmetric NSC division. (a) Time-lapse images of dividing NSCs in mouse embryonic neocortical slices. Neocortical NSCs in mouse embryos were transfected with expression plasmids for Dll1-EGFP and histone H2B (H2B)-mCherry byin uteroelectroporation at E13.5. After development of the embryos for an additional 15–19 hin utero, neocortical slices were prepared, cultured and subjected to time-lapse imaging of EGFP and mCherry fluorescence. Time is indicated relative to the timing of meta-anaphase transition. Broken lines indicate the ventricular surface. The cells are also shown inSupplementary Movie 4. Scale bar, 10 μm. (b) A typical example of dividing NSC sisters. In the left panel, (i) and (ii) indicate Dll1-inheriting and non-Dll1-inheriting sister cells, respectively. The cells are also shown inSupplementary Movie 5. The immunohistofluorescence staining of the corresponding cortical slice is shown in the right panels. (i) and (ii) denote the same sister cells indicated in the left panel. Scale bar, 10 μm. The position and orientation of each daughter cell in the ventricular zone of the cultured slice are also shown in low-magnification images (Supplementary Fig. S2). Figure 6: Dll1-EGFP moves to one daughter cell that becomes a neuronal progenitor during asymmetric NSC division. ( a ) Time-lapse images of dividing NSCs in mouse embryonic neocortical slices. Neocortical NSCs in mouse embryos were transfected with expression plasmids for Dll1-EGFP and histone H2B (H2B)-mCherry by in utero electroporation at E13.5. After development of the embryos for an additional 15–19 h in utero , neocortical slices were prepared, cultured and subjected to time-lapse imaging of EGFP and mCherry fluorescence. Time is indicated relative to the timing of meta-anaphase transition. Broken lines indicate the ventricular surface. The cells are also shown in Supplementary Movie 4 . Scale bar, 10 μm. ( b ) A typical example of dividing NSC sisters. In the left panel, (i) and (ii) indicate Dll1-inheriting and non-Dll1-inheriting sister cells, respectively. The cells are also shown in Supplementary Movie 5 . The immunohistofluorescence staining of the corresponding cortical slice is shown in the right panels. (i) and (ii) denote the same sister cells indicated in the left panel. Scale bar, 10 μm. The position and orientation of each daughter cell in the ventricular zone of the cultured slice are also shown in low-magnification images ( Supplementary Fig. S2 ). Full size image We also examined the behaviour of Dll1-EGFP in an in vitro culture of the adult SVZ by time-lapse imaging. A cell cycle indicator Fucci (mCherry-hGeminin (1/60)), which emits mCherry fluorescence during S/G2/M phases, was coexpressed with Dll1-EGFP to detect dividing cells easily before starting time-lapse imaging. We found that a large proportion of Dll1-EGFP + -dividing cells exhibited asymmetric Dll1-EGFP segregation between daughter cells (11/15 Dll1-EGFP + divisions) ( Fig. 7a ; Supplementary Movies 6 and 7 ). We then examined the fate of the non-Dll1-inheriting daughters by immunostaining with the adult NSC marker GFAP and found that a large proportion (7/11) of Dll1-negative daughter cells expressed GFAP ( Fig. 7b ). GFAP expression was also detected in daughter cells that did not inherit endogenous Dll1 puncta in the SVZ of adult brain ( Fig. 5d ; Supplementary Fig. S4 ). These results strongly support the notion that the non-Dll1-inheriting daughter cells were NSCs rather than transit-amplifying cells or differentiating neuroblasts. 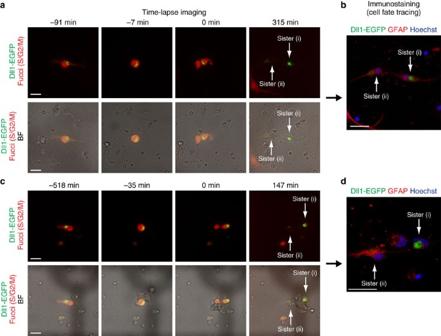Figure 7: Asymmetrical segregation of Dll1-EGFP in the adult SVZ culture. (a,c) Time-lapse images of dividing adult NSCs in the adult SVZ culture. Cultured adult SVZ NSCs were infected with recombinant retroviruses expressing Dll1-EGFP (green) and fucci probe mCherry-hGeminin (1/60) (red), which emits mCherry fluorescence in S/G2/M phases. The images of bright field (BF) were merged to the fluorescent images. Time is indicated relative to the timing of cytokinesis. (i) and (ii) indicate Dll1-inheriting and non-Dll1-inheriting sister cells, respectively. The cells inaandcare also shown inSupplementary Movies 6 and 7, respectively. (b,d) The cell fate of daughter cells inaandcwas shown inbandd, respectively. The adult NSC fate was verified by GFAP immunostaining after time-lapse imaging. (i) and (ii) denote the same sister cells indicated inaandc. Scale bar, 20 μm. Figure 7: Asymmetrical segregation of Dll1-EGFP in the adult SVZ culture. ( a , c ) Time-lapse images of dividing adult NSCs in the adult SVZ culture. Cultured adult SVZ NSCs were infected with recombinant retroviruses expressing Dll1-EGFP (green) and fucci probe mCherry-hGeminin (1/60) (red), which emits mCherry fluorescence in S/G2/M phases. The images of bright field (BF) were merged to the fluorescent images. Time is indicated relative to the timing of cytokinesis. (i) and (ii) indicate Dll1-inheriting and non-Dll1-inheriting sister cells, respectively. The cells in a and c are also shown in Supplementary Movies 6 and 7 , respectively. ( b , d ) The cell fate of daughter cells in a and c was shown in b and d , respectively. The adult NSC fate was verified by GFAP immunostaining after time-lapse imaging. (i) and (ii) denote the same sister cells indicated in a and c . Scale bar, 20 μm. Full size image These fate tracing data of embryonic and adult NSCs ( Figs 6 and 7 ) are consistent with the results of a previous study, showing that an increase in the amount of Dll1 promotes neuronal differentiation of neocortical NSCs, whereas its decrease inhibits this process [35] . These observations together support the notion that Dll1 is a fate determinant that segregates asymmetrically to one daughter cell during NSC mitosis, and that the cell that inherits Dll1 undergoes neuronal differentiation, whereas the non-Dll1-inheriting cell remains undifferentiated. Long-term maintenance of the undifferentiated and quiescent state, with the occasional exit from quiescence to produce neurons and glial cells, is a fundamental feature of adult NSCs. We have now revealed an essential role for Dll1 in the maintenance of quiescent NSCs in the adult mouse SVZ, as well as the asymmetric inheritance of Dll1 by one daughter cell during NSC division. Given the specific expression pattern of Dll1 in activated NSCs and transit-amplifying cells, as well as the location of Dll1-expressing cells in close proximity to quiescent NSCs, we propose that NSCs in the adult SVZ produce their own niche cells by asymmetric cell division. Although progeny of adult stem cells have recently been shown to become niche cells in other mammalian tissues such as hair follicle and intestine [46] , [47] , our findings are unique in suggesting that one daughter of an adult stem cell becomes a niche cell and supports its sister (stem) cell. The sister (niche) cell would be expected to reside next to the NSC immediately after division and might therefore be able effectively to provide a quiescence-inducing (and differentiation-inhibiting) signal during early G 1 phase of the cell cycle. Newborn progeny cells appear to modulate the behaviour of adult NSCs, given that elimination of rapidly proliferating progeny results in the activation of quiescent NSCs to support continuous neurogenesis in the adult SVZ [4] , [48] . Our finding that activated NSCs and transit-amplifying cells provide a signal that inhibits the proliferation of NSCs and subsequent neurogenesis might account, at least in part, for this phenomenon. This feedback mechanism might be beneficial for maintenance of the balance between NSCs and their progeny, which is key to ensuring that the brain is supplied with appropriate numbers of differentiated cells. A recent paper has shown that overexpression of EGFR in cells including transit-amplifying cells with the use of a Cnp promoter reduces Notch signalling in NSCs in a non-cell-autonomous manner and consequently decreases the number of NSCs, suggesting the existence of an additional feedback mechanism mediated by progeny cells [23] . The asymmetric distribution of endogenous Dll1 in both embryonic and adult NSCs at mitosis, as well as our real-time observation of the movement of Dll1-EGFP to one daughter cell during mitosis in neocortical slice cultures and adult SVZ cultures, suggests that Dll1 might be a long-sought determinant that establishes asymmetric cell fates for the two daughter cells of an NSC in the mammalian brain. Given that asymmetric distribution of Dll1 at mitosis was detected even in sparsely cultured NSCs, such asymmetry may be initiated by cell-intrinsic machinery. It is also possible that cell-extrinsic machinery further enhances (or biases) the asymmetry, given that the extent of asymmetric Dll1 distribution was found to be much higher in vivo than in vitro . It will be of interest to characterize the mechanisms responsible for the asymmetric distribution of Dll1, in particular with regard to the possible roles of centrioles [49] or molecules that have been associated with asymmetric NSC division (such as Par3, TRIM32, Dryk1 and EGFR) [18] , [19] , [20] , [21] . In Drosophila , Sara-positive vesicles that contain Delta move to one daughter cell in dividing sensory organ precursors [50] , although the function of Delta in these vesicles ( cis activation of Notch) appears to be opposite to the predicted function of Dll1 within the Dll1-expressing cells of the mouse SVZ ( cis inhibition and trans activation of Notch). It will be interesting, however, to investigate whether the molecules associated with the Drosophila Delta-containing vesicles (such as Sara) also contribute to Dll1 segregation in mammalian NSCs. A recent study on zebrafish forebrain development has shown that Mindbomb (Mib), a modulator of Notch ligand endocytosis, is asymmetrically segregated to a differentiating daughter cell during radial glial cell division and that asymmetrical localization of Mib is regulated by Par3 [51] . Even though the function of Par3 in the zebrafish brain (limiting progenitor self-renewal) seems to be different from the function in the mouse brain (promoting progenitor self-renewal) [18] , [52] , Mib or Par3 might also be involved in the Dll1 asymmetry in mouse NSC division. Quiescent NSCs undergo occasional activation to allow for the proliferation and differentiation that underlie the production of new neurons, but they must subsequently return (initialize) to the quiescent and undifferentiated state to avoid depletion of the stem cell pool. A recent study on adult zebrafish NSCs has shown that Notch activation can drive activated progenitors into quiescent NSCs [30] . We propose that asymmetric segregation of Dll1 can be considered a mechanism for ‘initialization’ of the stem cell state subsequent to NSC activation ( Fig. 8 ). Activation of NSCs in the adult SVZ is associated with the induction of Dll1 expression, which would be expected to promote their proliferation and differentiation. Given that Dll1 activates Notch in neighbouring cells ( trans activation) and inhibits Notch within the same cell ( cis inhibition), asymmetric segregation of Dll1 during NSC division would be expected to promote the activation of Notch signalling in the daughter NSC not only by providing a Dll1 signal to its sister cell but also by excluding Dll1 from the daughter NSC. Exclusion of Dll1 by asymmetric segregation, in addition to Notch activation by the Dll1-inheriting sister cell, thus results in the ‘initialization’ of the quiescent and undifferentiated state in activated NSCs. Activation of adult NSCs is also accompanied by the expression of Ascl1, which promotes the proliferation and differentiation of NSCs [53] . Given that the function and expression of Ascl1 are antagonized by Notch signalling, exclusion of Dll1 might also result in inactivation of Ascl1 in a daughter NSC. Furthermore, because transcription of Dll1 is positively regulated by Ascl1 [54] , inactivation of Ascl1 function by Dll1 exclusion might further suppress Dll1 transcription. Such a feedback system might reinforce the successful return (initialization) of an activated NSC to the stem cell state. According to our model, a long-term disruption of the initialization of stem cell state may cause a depletion of NSC pool and NSC progeny. However, we could not show this because of an expansion of NSCs without the Dll1 gene deletion (‘escapers’), which can happen when a gene essential for NSC maintenance is deleted incompletely [55] . 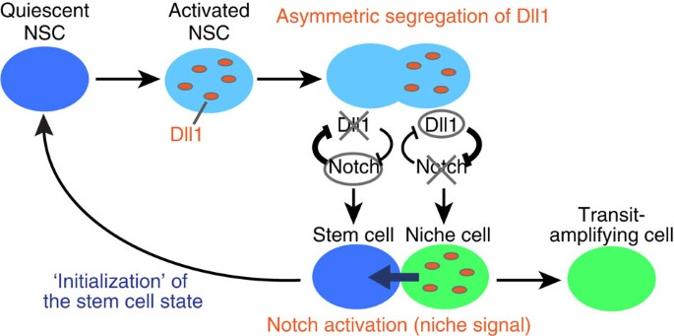Figure 8: Model for initialization of the stem cell state subsequent to NSC activation and asymmetric Dll1 segregation. Activation of quiescent NSC is associated with the induction of Dll1 expression. After asymmetric Dll1 segregation, Notch signalling of non-Dll1-inheriting sister cell is activated through both the exclusion ofcis-inhibitory Dll1 and the niche signal (transactivation) from Dll1-inheriting sister cell, which ‘initializes’ the non-Dll1-inheriting sister into the quiescent stem cell state. Figure 8: Model for initialization of the stem cell state subsequent to NSC activation and asymmetric Dll1 segregation. Activation of quiescent NSC is associated with the induction of Dll1 expression. After asymmetric Dll1 segregation, Notch signalling of non-Dll1-inheriting sister cell is activated through both the exclusion of cis -inhibitory Dll1 and the niche signal ( trans activation) from Dll1-inheriting sister cell, which ‘initializes’ the non-Dll1-inheriting sister into the quiescent stem cell state. Full size image Then, how do quiescent NSCs become activated? In the basal state, it appears plausible to assume a mechanism (‘timer’) that regulates the activation of NSCs at a low frequency. The accumulation of Dll1 might be regulated by this timer, or, alternatively, the accumulation of Dll1 itself might be a timer that induces activation of NSCs after it has exceeded a threshold. Activation of NSCs in the adult brain is also induced in association with various physiological and pathological conditions. The transcription of Dll1 is regulated in other systems by the signalling pathways, such as the Wnt and STAT pathways [56] , [57] , [58] , which have been implicated in the activation of NSCs in the adult brain. The possible roles of Dll1 induction in various contexts of NSC activation thus warrant further investigation. The distribution of Dll1 thus appears key to an understanding of NSC maintenance and might affect aging and tumorigenesis when altered during adulthood. Further characterization of the regulation of Dll1 expression and distribution during mitosis may provide insight into NSC regulation in stem cell biology and regenerative medicine. Mice Adult (2–6-month old) ICR mice (Clea Japan), C57BL6 mice or Dll1 cKO mice were used for immunohistofluorescence analysis, administration of thymidine analogues, Ara-C infusion and primary adult SVZ cultures. ICR mouse embryos (Clea Japan) were used for immunohistofluorescence analysis as well as for preparation of primary NSC cultures and neocortical slice cultures. Dll1 cKO mice were obtained by crossing Dll1 f/f mice [40] and NesCreERT2 mice (kindly provided by R. Kageyama); for activation of CreERT2, tamoxifen (Sigma; 200 μl of a 20 mg ml −1 solution in sunflower oil) was injected intraperitoneally 1–3 times (one injection per day). All mice were maintained according to protocols approved by the Animal Care and Use Committee of the University of Tokyo. Expression constructs and antibodies The plasmids pcDNA5/TO-histone H2B-mCherry, Fucci probe mCherry-hGeminin (1/60), vesicular stomatitis virus G-expressing vector and pMXs vector were kindly provided by Y. Watanabe, A. Miyawaki, H. Song and T. Kitamura, respectively. For construction of an expression vector for mouse Dll1 tagged at its COOH terminus with EGFP (Dll1-EGFP), the entire Dll1-coding sequence without the stop codon was inserted into pEGFP-N1 (Clontech). For retrovirus induction, Dll1-EGFP and mCherry-hGeminin (1/60) were inserted to pMXs vector to yield pMXs-Dll1-EGFP and pMXs-mCherry-hGeminin (1/60). Antibodies used for immunofluorescence analysis are listed in Supplementary Information . For a more detailed description, see Supplementary Methods in Supplementary Information . Immunofluorescence analysis For immunohistofluorescence staining of coronal brain sections, brains were fixed with 4% paraformaldehyde in PBS at 4 °C for 1–4 h. After equilibration with 30% (w/v) sucrose in PBS, the fixed brains were embedded in OCT compound (Tissue TEK) and frozen. Coronal cryosections (10–20 μm thickness) were exposed to TBS containing 0.1–0.5% Triton X-100 and 2% donkey serum (blocking buffer) for 2 h at room temperature (RT), and incubated first overnight at 4 °C with primary antibodies in blocking buffer and then 2 h at RT with Alexa Fluor-conjugated secondary antibodies in blocking buffer. For staining with the antibody to NICD, we used target retrieval solution (Dako) for antigen retrieval and a tyramide signal amplification kit (Molecular Probes) for signal enhancement. We used citrate buffer for antigen retrieval in staining of thymidine analogues. Antigen retrieval was performed by autoclave treatment of sections for 5–10 min at 105 °C. To obtain an en-face view of the ventricular surface, we stained whole-mount preparations of the dissected NCX. Whole-mount preparations were fixed with 4% paraformaldehyde at 4 °C for 1–6 h, exposed to blocking buffer and incubated first overnight at 4 °C with primary antibodies in blocking buffer and then either overnight at 4 °C or for 6–10 h at RT with Alexa Fluor-conjugated secondary antibodies in blocking buffer. For immunocytofluorescence staining of embryonic NSC cultures and adult SVZ cultures, cells were fixed with 4% paraformaldehyde in PBS for 10–20 min, permeabilized with 0.1–0.2% Triton X-100 for 10–20 min, exposed to PBS containing 3–5% BSA for 30 min, incubated with primary antibodies overnight and then with secondary antibodies for 30–60 min, and mounted in Mowiol (Calbiochem). Fluorescence images were obtained with a laser confocal microscope (Leica TCS-SP5 or Zeiss LSM510). Images were processed with the use of LAS AF (Leica), Photoshop CS (Adobe), QuickTime Pro (Apple) and Image J (US National Institutes of Health) software. Simultaneous detection of mRNA and protein To detect Dll1 mRNA and protein simultaneously, cryosections were first subjected to immunohistofluorescence analysis. After labelling Dll1 proteins using anti-Dll1 antibody with Alexa Fluor-labelled secondary antibodies, sections were fixed with 4% paraformaldehyde for 10 min at RT and then subjected to subsequent fluorescence in situ hybridization. The digoxigenin (DIG)-labelled antisense riboprobe for detecting mouse Dll1 corresponds to nucleotides 907–1851 (NM_007865.3). After paraformaldehyde fixation, sections were exposed to PBS, treated with proteinase K (2 μg ml −1 ) for 10 min at RT, followed by incubation in 4% paraformalidehyde for 5 min at RT and washing with PBS. Then, the sections were treated with TEA buffer (100 mM triethanolamine and 0.2% acetic acid) for 10 min at RT, washed with PBS, pre-hybridized with hybridization solution (50% formamide, 5 × saline-sodium citrate (SSC), 5 × denhardts, 200 μg ml −1 salmon sperm DNA and 1 mg ml −1 yeast RNA) for 1 h at 50–60 °C and incubated with hybridization solution containing DIG-labelled riboprobes at 50–60 °C overnight. Then, they were washed with 1 × SSC for 15 min and 0.1 × SSC for 20 min twice at 50–60 °C, PBS containing 0.1% tween20 for 5 min at RT and PBS for 5 min twice at RT, blocked with blocking buffer (PBS containing 5% BSA) for 1 h at RT and then incubated with blocking buffer containing anti-DIG POD (Roche) for 2 h at RT. The sections were washed with PBS twice at RT and then incubated with Alexa Fluor-labelled tyramide (Molecular Probes) for 10 min at RT. Then the sections were washed with PBS containing 0.1% tween20 twice, incubated with Hoechst 33342 for 30min at RT, washed with PBS twice and mounted into Mowiol. Administration of thymidine analogues For identification of LRCs, IdU (Sigma) was injected daily and intraperitoneally (57.5 mg kg −1 ) for the number of days indicated. Mice were killed at the indicated number of days after the last IdU injection. For labelling of rapidly dividing cells, mice were killed 1 h after administration of a single intraperitoneal dose (42.5 mg kg −1 ) of CldU (Sigma). Cells positive for IdU or CldU were detected by immunostaining. Ara-C infusion Ara-C (2%; Sigma) in PBS was infused for 6 days onto the surface of the adult mouse brain with the use of a miniosmotic pump (Alzet; model 1007D). Cannulas (Alzet; Brain infusion kit III) were implanted in the lateral ventricle (anterior: 0 mm, lateral: 1.1 mm and depth: 2 mm relative to bregma and the surface of the brain) [4] . One day after pump removal, the mice were killed for immunostaining of brain sections. In utero electroporation and time-lapse imaging E13.5 ICR embryos (E1 was defined as 12 h after detection of the vaginal plug) were subjected to electroporation in utero with expression vectors for Dll1-EGFP and histone H2B tagged with mCherry. The uterine horn was returned to the abdominal cavity, and the embryos were allowed to continue development for 15–19 h. The embryos were then collected, and cortical slices were prepared and cultured in collagen gels with enriched culture medium. Time-lapse images were obtained by confocal microscopy (TCS-SP5; Leica). For determination of the fate of daughter cells after NSC division, cortical slices were fixed with 4% paraformaldehyde immediately after time-lapse imaging and subjected to immunostaining. For a more detailed description, see Supplementary Methods in Supplementary Information . Primary embryonic NSC culture We used primary embryonic NSCs as a model of adult SVZ NSCs. Even though there are a number of differences between embryonic NSCs and adult NSCs, embryonic NSCs can still be considered as a good model for adult NSCs because it has been reported that embryonic NSCs (radial glial cells) are the origin of adult NSCs, and there are considerable similarities between them, such as cell type-specific morphology (junctional complexes formed by the apical endings), the apical–basal polarity and the expression of cell type-specific markers (for example, Sox2, Nestin and RC1) [59] , [60] . Cells were prepared from the dorsal cerebral cortex of ICR mouse embryos at E11.5, and an NSC-enriched population was obtained by neurosphere culture [35] . The cultured NSCs were subjected to immunocytofluorescence staining. Primary adult SVZ culture SVZs were dissected from the lateral wall of the lateral ventricle of adult (2 months) ICR mice and then dissociated using Nerve-Cell Culture System/Dissociation Solution (Sumitomo Bakelite). For immunocytofluorescence analysis, dissociated cells were cultured for 3 days and then subjected to immunofluorescence analysis. For time-lapse imaging, cells were mixed with recombinant retroviruses expressing Dll1-EGFP and mCherry-hGeminin (1/60) for 16–20 h, then incubated with fresh medium for 18–30 h. Time-lapse images were acquired using a Cell Voyager CV1000 (Yokogawa). After time-lapse imaging, the cultured cells were subjected to immunocytofluorescence staining to determine the fate of daughter cells. For a more detailed description, see Supplementary Methods in Supplementary Information . Statistical analysis Quantitative data in Figs 2 and 3 are means±s.e.m. of values (the number of cells in an area of 1 mm width along the ventricular surface) from 6–12 sections of one brain of each genotype as indicated in each figure legend, and similar results were obtained for a total of three brain pairs in independent experiments. Corresponding sections are obtained from nearly the same anterior–posterior position of the SVZ. Quantitative immunostaining data in Fig. 1 and in the text are means±s.d. for three brains. The experiments were repeated at least three times with similar results. To quantify the number of LRCs residing very close to Dll1 + cells ( Fig. 1c ), we defined ‘10-μm distance between nuclei’ as two cells that reside next to each other. Asymmetric Dll1 distribution was defined as a >3-fold difference in Dll1-immunostaining intensity between daughter cells. Data were compared between groups with the unpaired Student’s t -test. A P -value of <0.05 was considered statistically significant. How to cite this article: Kawaguchi, D. et al. Dll1 maintains quiescence of adult neural stem cells and segregates asymmetrically during mitosis. Nat. Commun. 4:1880 doi: 10.1038/ncomms2895 (2013).